The parasiteEntamoeba histolyticaexploits the activities of human matrix metalloproteinases to invade colonic tissue Intestinal invasion by the protozoan parasite Entamoeba histolytica is characterized by remodelling of the extracellular matrix (ECM). The parasite cysteine proteinase A5 (CP-A5) is thought to cooperate with human matrix metalloproteinases (MMPs) involved in ECM degradation. Here, we investigate the role CP-A5 plays in the regulation of MMPs upon mucosal invasion. We use human colon explants to determine whether CP-A5 activates human MMPs. Inhibition of the MMPs’ proteolytic activities abolishes remodelling of the fibrillar collagen structure and prevents trophozoite invasion of the mucosa. In the presence of trophozoites, MMPs-1 and -3 are overexpressed and are associated with fibrillar collagen remodelling. In vitro , CP-A5 performs the catalytic cleavage needed to activate pro-MMP-3, which in turn activates pro-MMP-1. Ex vivo , incubation with recombinant CP-A5 was enough to rescue CP-A5-defective trophozoites. Our results suggest that MMP-3 and/or CP-A5 inhibitors may be of value in further studies aiming to treat intestinal amoebiasis. The enteropathogen parasite Entamoeba histolytica infects 10% of the world’s population [1] and causes ~100,000 deaths per year [2] . Intestinal amoebiasis is characterized by severe colitis and bloody dysentery. The development of a colon explant-based model of human amoebiasis [3] has enabled characterization of the sequence of early events leading to intestinal amoebiasis. Invasion of the human colonic mucosa by E. histolytica is characterized by an acute pro-inflammatory reaction. Indeed, induction of the secretion of cytokines (particularly interleukin (IL)-1β, IL-6, IL-8, interferon-γ and tumour necrosis factor (TNF)-α [3] ) appears to be the central factor in the genesis of disease. Furthermore, perturbation of the extracellular matrix (ECM) is required for E. histolytica to invade the lamina propria [4] . Cysteine proteinases are major virulence factors in trophozoites [5] , [6] , [7] . The cysteine proteinase A5 (CP-A5) interacts directly with integrins at the surface of human colon epithelial cells and induces the secretion of pro-inflammatory cytokines (including TNF-α and IL-1β; ref. 8 ). Thus, trophozoites epigenetically silenced for CP-A5 (that is, CP-A5 negative) fail to trigger a host inflammatory response or induce the collagen remodelling required for invasion of the lamina propria [3] , [4] . Interestingly, the matrix metalloproteinase (MMP) genes are known to be transcriptionally responsive to several factors, including cytokines such as TNF-α and IL-1β (ref. 9 )—both of which are inflammatory markers of intestinal amoebiasis and are strongly induced by CP-A5. Furthermore, it has been reported that the MMPs-1 and -3 genes were overexpressed in patients suffering from intestinal amoebiasis [10] . It is well known that MMPs are responsible for degrading the ECM in connective tissue [11] . Based on substrate specificity and structural homology, 24 MMPs have been identified and classified as collagenases (MMPs-1, -8, -13 and -18), gelatinases (MMPs-2 and -9), stromelysins (MMPs-3, -7, -10 and -11), elastase (MMP-12), membrane-type MMPs (MMPs-14, -15, -16, -17, -24 and -25) and others (MMPs-19, -20, -23, -26, -27 and -28; ref. 11 ). All MMPs have a similar domain structure, with a predomain required for secretion, a prodomain maintaining latency and an active catalytic region that contains the zinc-binding active site. The MMPs are secreted as latent enzymes and become activated by the action of other MMPs or serine protease that cleave a peptide bond within the prodomain [9] . For instance, MMP-3 has been shown to be an important activator of other MMPs, including MMP-1 (ref. 12 ) (one of only three MMPs, along with MMPs-8 and -13, known to initiate the intrahelix cleavage of triple-helix collagen [13] , [14] ). The enzymatic activity of MMPs is regulated by tissue endogenous inhibitors of MMPs (TIMPs), which act by forming a 1:1 complex with the highly conserved zinc-binding site of MMPs. The resulting [MMP-TIMP] complex is inactive and unable to bind substrate. In previous work [4] , we demonstrated that CP-A5 cooperates with human tissue factors during trophozoite invasion of the intestinal mucosa. Given that CP-A5 induces TNF-α and IL-1β secretion (which in turn can induce MMP expression), we decided to investigate the role of the MMPs’ enzymatic activities during intestinal amoebiasis. Since most of the MMPs are released as inactive pro-MMPs, we hypothesized that CP-A5 might directly activate pro-MMPs. Here we study the role of the MMPs’ enzymatic activity and examine the expression pattern and the localization of MMPs-1, -3, -7 and -9 in human colonic explants challenged with E. histolytica . We probed the activation of MMPs by CP-A5 in vitro by using recombinant CP-A5 and purified pro-MMPs-1 and -3. Our data indicate that CP-A5 can directly convert pro-MMP-3 into its mature form, which in turn activates pro-MMP-1. Finally, we propose that the CP-A5 has the following two functions during intestinal invasion: (i) the indirectly triggering of MMP production and release through inflammatory cytokine induction, and (ii) directly catalytic cleavage of pro-MMP-3 and thus conversion into active MMP-3. Together, these processes are involved in the ECM remodelling required for tissue invasion. Human MMP activity is required for intestinal invasion We first sought to determine whether human MMP enzymatic activities are involved in intestinal tissue invasion by E. histolytica. We incubated E. histolytica trophozoites on human colon explants for 7 h in the presence or absence of marimastat (a broad-spectrum, low-molecular-weight MMP inhibitor with an IC 50 ranging from 2 to 200 nM for purified enzymes [15] ) ( Fig. 1 ). Marimastat is highly specific to human metalloproteinase belonging to the MA clan, families M10 and M12, which are not present in E. histolytica . The colon fragments were fixed for histological analysis, and longitudinal tissue sections were prepared and analysed ( Fig. 1 ). We controlled the effect of marimastat on E. histolytica by pre-incubated trophozoites with marimastat 30 min prior the incubation on human colon tissue. Treatment with marimastat alone had no effect on the trophozoites’ invasiveness, since marimastat-treated trophozoites subsequently invaded the tissue to the same extent as wild-type (WT) trophozoites [3] , [4] ( Fig. 1a ). In contrast, trophozoites challenged for invasion of marimastat-treated tissue were able to remove and detach epithelial cells but failed to invade the lamina propria. Quantification of tissue invasion for each condition in four biological replicates is shown in Fig. 1b . 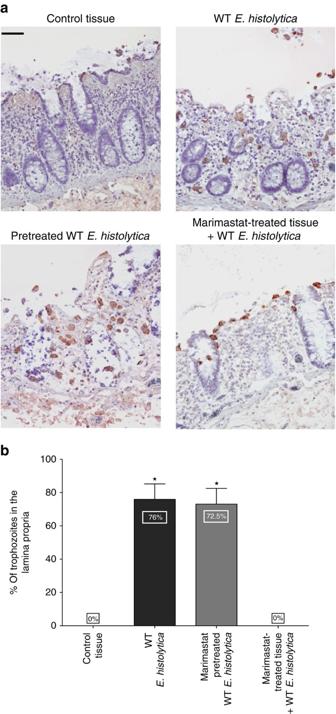Figure 1: Inhibition of MMP activity abolishes colonic mucosa invasion. Human colon explants were incubated for 7 h withE. histolytica, fixed and included in paraffin. Tissue sections were then processed for immunohistochemistry. (a) Trophozoites were immunohistochemically stained for Gal/GalNAc lectin (brown cells) and tissue cells counterstained with haematoxylin–eosin. The upper left panel shows the standard tissue architecture of a colon explant where epithelial cells are revealed in magenta and delineate the intestinal crypts. In the presence of WT trophozoites (upper right panel), the tissue architecture was altered and trophozoites were found in the lamina propria. When trophozoites were treated with marimastat (lower left panel), there is no changes in the invasive phenotype and the architecture of the colonic mucosa was altered. In the absence of MMP activities (that is, in the presence of marimastat), trophozoites detached the epithelium but failed to invade the lamina propria (lower right panel). One representative image of the four experiments performed is shown. Scale bar, 50 μm.n=4. (b) For each condition, trophozoites present in the lamina propria were quantified. Data are shown as mean and the s.d. The data are from four independent experiments (n=4). Nonparametric Mann–Whitney test was performed; *P<0.05. Figure 1: Inhibition of MMP activity abolishes colonic mucosa invasion. Human colon explants were incubated for 7 h with E. histolytica , fixed and included in paraffin. Tissue sections were then processed for immunohistochemistry. ( a ) Trophozoites were immunohistochemically stained for Gal/GalNAc lectin (brown cells) and tissue cells counterstained with haematoxylin–eosin. The upper left panel shows the standard tissue architecture of a colon explant where epithelial cells are revealed in magenta and delineate the intestinal crypts. In the presence of WT trophozoites (upper right panel), the tissue architecture was altered and trophozoites were found in the lamina propria. When trophozoites were treated with marimastat (lower left panel), there is no changes in the invasive phenotype and the architecture of the colonic mucosa was altered. In the absence of MMP activities (that is, in the presence of marimastat), trophozoites detached the epithelium but failed to invade the lamina propria (lower right panel). One representative image of the four experiments performed is shown. Scale bar, 50 μm. n =4. ( b ) For each condition, trophozoites present in the lamina propria were quantified. Data are shown as mean and the s.d. The data are from four independent experiments ( n =4). Nonparametric Mann–Whitney test was performed; * P <0.05. Full size image Human MMP activity is responsible for collagen remodelling We had previously shown that intestinal invasion by E. histolytica requires collagen fibre remodelling [4] . Thus, we next looked at whether the inhibition of intestinal invasion in the presence of marimastat was correlated with a defect in collagen remodelling (as a consequence of MMP inhibition). We visualized the tissue’s fibrillar collagen network with second-harmonic imaging microscopy (SHIM) ( Fig. 2 ). Trophozoites (WT or marimastat-pretreated trophozoites) were incubated with human tissue explants in the presence or absence of marimastat. After 2 h of invasion in the presence of marimastat, no remodelling of the fibrillar collagen structures was observed. The fibrillar collagen architecture was not altered, with the characteristic collagen rings around the crypts and a structured collagen meshwork extending into the lamina propria (as observed in the control tissue) [4] . However, in the absence of marimastat, WT trophozoites and marimastat-pretreated trophozoites induced strong remodelling of the collagen network. The remodelled network was characterized by wavy collagen bundles and collapsing crypts, as previously described [4] . Further, we verified that marimastat has no effect on the collagenolytic activity of parasites ( Fig. 3 ). These observations strongly suggest that human MMPs are involved in collagen remodelling upon intestinal invasion by E. histolytica . 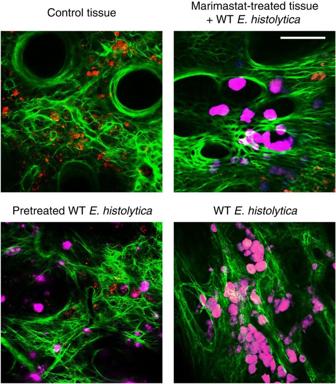Figure 2: Lack of human MMP activity preserves the fibrillar collagen network. Human colon explants were incubated withE. histolyticaand imaged with multiphoton microscopy. Fibrillar collagen structures appeared in green (second harmonic generation (SHG) signal), whereas endogenous cells appear in red (autofluorescence signal). The upper left panel shows the typical collagen collagen rings around the crypts and a structured collagen meshwork extending into the lamina propria. In the presence of WT trophozoites (purple) and marimastat-pretreated trophozoites, the fibrillar collagen network was drastically altered (lower right and left panels). However, in the absence of human MMP activities (that is, in the presence of marimastat), fibrillar collagen structures were still intact (upper right panel). One representative image of the four experiments performed is shown. Scale bar, 50 μm.n=4. Figure 2: Lack of human MMP activity preserves the fibrillar collagen network. Human colon explants were incubated with E. histolytica and imaged with multiphoton microscopy. Fibrillar collagen structures appeared in green (second harmonic generation (SHG) signal), whereas endogenous cells appear in red (autofluorescence signal). The upper left panel shows the typical collagen collagen rings around the crypts and a structured collagen meshwork extending into the lamina propria. In the presence of WT trophozoites (purple) and marimastat-pretreated trophozoites, the fibrillar collagen network was drastically altered (lower right and left panels). However, in the absence of human MMP activities (that is, in the presence of marimastat), fibrillar collagen structures were still intact (upper right panel). One representative image of the four experiments performed is shown. Scale bar, 50 μm. n =4. 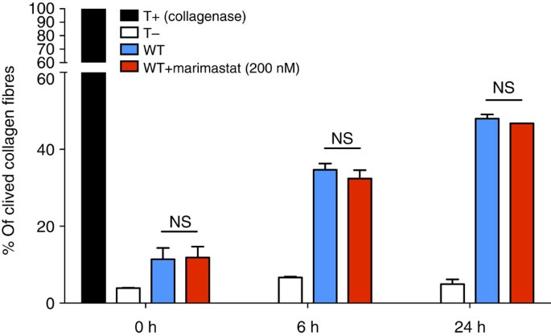Figure 3: Marimastat treatment does not affectE. histolyticacollagenase activity. Trophozoites treated with or without marimastat were incubated in a three-dimensional matrix of fibrillar collagen I. The release of fluorescence from soluble fluorescein isothiocyanate-labelled collagen was measured by spectrofluorescence and quantified. No significant difference in cleaved collagen fibres was observed in the presence of marimastat as compared with the untreated WT strain. Total degradation of the matrix usingClostridiumcollagenase was obtained with 7 U ml−1at 37 °C after 6 h of incubation. Data are shown as mean and the s.e.m. The data are from four independent experiments (n=4). Nonparametric Mann–Whitney test was performed. NS, not significant;P≧0.05). Full size image Figure 3: Marimastat treatment does not affect E. histolytica collagenase activity. Trophozoites treated with or without marimastat were incubated in a three-dimensional matrix of fibrillar collagen I. The release of fluorescence from soluble fluorescein isothiocyanate-labelled collagen was measured by spectrofluorescence and quantified. No significant difference in cleaved collagen fibres was observed in the presence of marimastat as compared with the untreated WT strain. Total degradation of the matrix using Clostridium collagenase was obtained with 7 U ml −1 at 37 °C after 6 h of incubation. Data are shown as mean and the s.e.m. The data are from four independent experiments ( n =4). Nonparametric Mann–Whitney test was performed. NS, not significant; P ≧ 0.05). Full size image MMPs-1 and -3 genes are upregulated upon intestinal invasion Given that the CP-A5-silenced strain of E. histolytica is not able to induce a pro-inflammatory response [3] or collagen remodelling [4] , we sought to determine whether CP-A5 was involved in human MMP expression during intestinal invasion. We examined the expression of MMPs-1 and -3 (which are known to be expressed during intestinal amoebiasis [10] ) and MMPs-7 and -9 (colon cancer markers [16] , [17] ) using a quantitative real-time PCR (qRT–PCR) assay of cDNA obtained after reverse transcription of mRNA extracted from formalin-fixed, paraffin-embedded (FFPE) tissue ( Fig. 4 ). The assays evidenced the specific upregulation of MMP-1 (fold change: 4.6±s.e.m. 0.79) and MMP-3 (fold change: 4.0±s.e.m. 0.75) gene expression upon intestinal invasion, which is consistent with previous results obtained for patient biopsies [10] . Human colonic mucosa incubated for 7 h with CP-A5-silenced trophozoites did not show a significant increase in MMP-1 (fold change: 1.6±s.e.m. 0.68) and MMP-3 (fold change: 1.1±s.e.m. 0.12) mRNA production, suggesting that CP-A5 is indeed essential for inducing MMPs-1 and -3 transcription. Similar observations were made when trophozoites were challenged for invasion of marimastat-treated tissue; expression of the MMP-1 gene (fold change: 0.98±s.e.m. 0.16) and the MMP-3 gene (fold change: 1.2±s.e.m. 0.08) was not significantly modulated. There was no evidence of MMP-7 or -9 mRNA production-confirming that MMPs-1 and -3 are specifically induced by E. histolytica invasion. 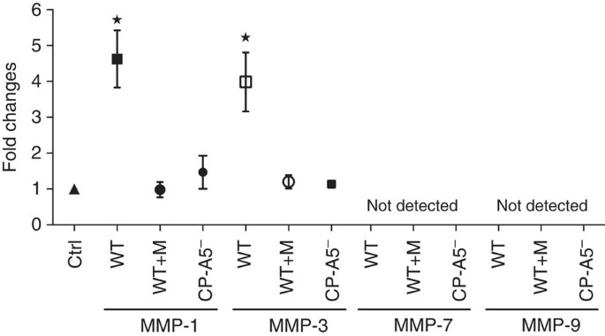Figure 4: MMPs-1 and -3 genes are overexpressed upon colon invasion byE. histolytica. Human colon explants were incubated with WT trophozoites (± marimastat) and CP-A5-silenced trophozoites for 7 h. MMPs-1, -3, -7 and -9 gene expression were analysed by qRT–PCR and compared with control tissue (in the absence of trophozoites). MMPs-1 and -3 were both overexpressed in the presence of the WT strain, whereas marimastat tissue treatment or CP-A5-silenced trophozoites failed to induce significant expression of MMPs-1 and -3 genes. Expression of the MMPs-7 and -9 genes was never detected. Results are shown as mean and the s.e.m. The data are from seven independent experiments (n=7). Nonparametric Mann–Whitney test was performed. *P<0.05. Figure 4: MMPs-1 and -3 genes are overexpressed upon colon invasion by E. histolytica . Human colon explants were incubated with WT trophozoites (± marimastat) and CP-A5-silenced trophozoites for 7 h. MMPs-1, -3, -7 and -9 gene expression were analysed by qRT–PCR and compared with control tissue (in the absence of trophozoites). MMPs-1 and -3 were both overexpressed in the presence of the WT strain, whereas marimastat tissue treatment or CP-A5-silenced trophozoites failed to induce significant expression of MMPs-1 and -3 genes. Expression of the MMPs-7 and -9 genes was never detected. Results are shown as mean and the s.e.m. The data are from seven independent experiments ( n =7). Nonparametric Mann–Whitney test was performed. * P <0.05. Full size image Localization of MMPs-1 and -3 in the colonic mucosa In order to localize the tissue compartment within which MMPs-1 and -3 are produced upon amoebic invasion, we performed an immunofluorescence analysis of histological tissue sections ( Fig. 5 ). WT and CP-A5-silenced trophozoites were incubated with human tissue explants and compared with control explants. After a 7-h incubation, the control tissue was still intact and well organized; MMPs-9 and -1 were not detected and few of the shed epithelial cells stained positive for MMP-3. The same observations were made in the presence of the CP-A5-silenced mutant. 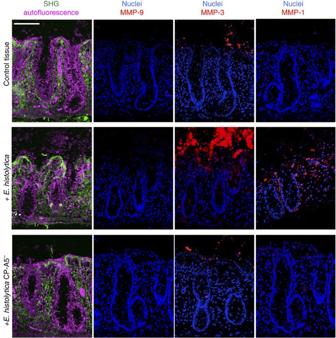Figure 5: Localization of MMPs -1, -3 and -9 upon colon invasion byE. histolytica. Human colon explants were incubated with WT and CP-A5-silenced trophozoites for 7 h fixed and included in paraffin. Tissue sections were image by two-photon microscopy. Autofluorescence (pink) and SHG (green) signals were acquired in order to visualize the colon explant’s organization (left column). MMPs-1, -3 and -9 were revealed by immunofluorescence (red). In the control tissue, neither MMP-9 nor MMP-1 was detected, but slight expression of MMP-3 was observed in epithelial cells. In the presence of WT trophozoites, a strong increase in MMPs-1 and -3 proteins was observed. MMP-3 was mainly expressed in epithelial cells, whereas MMP-1 was located in the lamina propria and on the basal side of the crypts. In the presence of the CP-A5-silenced strain, the pattern of MMPs-1 and -3 localization was the same as in the control condition. MMP-9 was never detected under any of the tested conditions. One representative image of the four experiments performed is shown. Scale bar, 50 μm,n=4. Figure 5: Localization of MMPs -1, -3 and -9 upon colon invasion by E. histolytica . Human colon explants were incubated with WT and CP-A5-silenced trophozoites for 7 h fixed and included in paraffin. Tissue sections were image by two-photon microscopy. Autofluorescence (pink) and SHG (green) signals were acquired in order to visualize the colon explant’s organization (left column). MMPs-1, -3 and -9 were revealed by immunofluorescence (red). In the control tissue, neither MMP-9 nor MMP-1 was detected, but slight expression of MMP-3 was observed in epithelial cells. In the presence of WT trophozoites, a strong increase in MMPs-1 and -3 proteins was observed. MMP-3 was mainly expressed in epithelial cells, whereas MMP-1 was located in the lamina propria and on the basal side of the crypts. In the presence of the CP-A5-silenced strain, the pattern of MMPs-1 and -3 localization was the same as in the control condition. MMP-9 was never detected under any of the tested conditions. One representative image of the four experiments performed is shown. Scale bar, 50 μm, n =4. Full size image However, upon invasion by WT E. histolytica , massive MMP-3 expression was observed in the epithelial cells. A western blot analysis of tissue sections showed a 5.3-fold increase in the activated form of MMP-3 in the presence of WT trophozoites, when compared with CP-A5-silenced trophozoites ( Fig. 6a ). This result suggests that WT trophozoites directly activate pro-MMP-3 into its mature form (possibly through CP-A5). MMP-1 was detected in stromal cells and along the crypts in regions where fibrillar collagen is known to be present [4] . Given that MMP-1 is known to initiate the intrahelix cleavage of triple-helix collagen [13] , [14] , we used immunofluorescence microscopy to check for intrahelix-cleaved collagen fibres ( Fig. 6b,c ). The presence of intrahelix-cleaved collagen fibres in the vicinity of the accumulated MMP-1 suggests that the latter is likely to be active. Taken as a whole, these observations suggest that CP-A5 is important for MMPs-1 and -3 expression and activation in the human colonic mucosa. 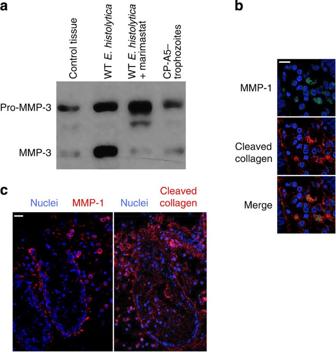Figure 6: Mature MMPs-1 and -3 are present during colonic invasion byE. histolytica. Human colon explants were incubated with WT and CP-A5-silenced trophozoites for 7 h, fixed and included in paraffin. (a) Western blot analysis of MMP-3 was performed from total protein extract obtained from FFPE tissue. Mature MMP-3 was only observed in the presence of WT trophozoites. (b,c). Immunofluorescence analysis of MMP-1 and collagenase cleavage type I and II collagen fibres was performed from FFPE tissue section. Collagenase-cleaved collagen type I and II is observed in the vicinity of MMP-1. Scale bars, 10 μm. Figure 6: Mature MMPs-1 and -3 are present during colonic invasion by E. histolytica . Human colon explants were incubated with WT and CP-A5-silenced trophozoites for 7 h, fixed and included in paraffin. ( a ) Western blot analysis of MMP-3 was performed from total protein extract obtained from FFPE tissue. Mature MMP-3 was only observed in the presence of WT trophozoites. ( b , c ). Immunofluorescence analysis of MMP-1 and collagenase cleavage type I and II collagen fibres was performed from FFPE tissue section. Collagenase-cleaved collagen type I and II is observed in the vicinity of MMP-1. Scale bars, 10 μm. Full size image CP-A5 is able to cleave pro-MMP-3 into mature MMP-3 Given that MMPs can be activated by other proteases, we next sought to determine whether CP-A5 is involved in the proteolytic activation of MMPs-1 and -3. To this end, we produced two recombinant proteins; a WT pro-CP-A5 and an inactive mutant in which the cysteine 119 in the catalytic site was mutated into a serine. After activation of the pro-WT-r-CP-A5 and pro-C119S-r-CP-A5 ( Supplementary Fig. 1A ), their enzymatic activities were measured using a specific fluorescent substrate for cysteine proteases Z-Arg-Arg-4-amino-7-methylcoumarin (ZRR-AMC) ( Fig. 7a ). We used purified cathepsin as a positive control for cysteine protease activity and the substrate ZRR-AMC alone was used as a negative control. After a 2-h incubation, we observed a significant increase in the enzymatic activity of WT-r-CP-A5 (specific activity: 72.7 μmol min −1 mg −1 ), when compared with C119S-r-CP-A5 (specific activity: 31 μmol min −1 mg −1 ). This result confirms that the C119S mutation indeed affects the enzymatic activity of CP-A5, although the activated r-CP-A5-C119S does have more protease activity than the non-activated C119S-r-CP-A5 ( Fig. 7a ). 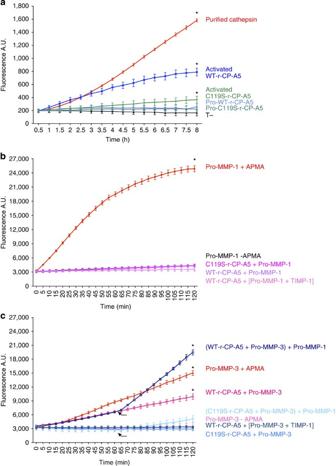Figure 7: Mature WT-CP-A5 activates pro-MMP-3 but not pro-MMP-1. (a) We evaluated the cysteine protease activity of WT-r-CP-A5 and C119S-r-CP-A5 using a specific fluorescence substrate (ZRR-AMC). No cysteine protease activity was observed with immature proteases (pro-WT-r-CP-A5 and pro-C119S-r-CP-A5). The WT-r-CP-A5 possesses proteolytic activity but this was very low in the C119S mutant. (b,c) We measured MMP activities using the MMP-specific substrate FS-6 specific. (b) Pro-MMP-1 and [MMP-1:TIMP-1] complex was incubated with either WT-r-CP-A5 or C119S-r-CP-A5 but was never activated. (c) Pro-MMP-3 was specifically activated by the mature WT-CP-A5. This activation required the enzymatic activity of CP-A5. Interestingly, MMP-3 activated by WT-r-CP-A5 can in turn convert pro-MMP-1 (arrow heads) into its mature form. Results are shown as mean and the s.d. Data are shown as mean and the s.d. The data are from six independent experiments,n=6. Nonparametric Mann–Whitney test was performed, *P<0.05. A.U.: arbitrary units. Figure 7: Mature WT-CP-A5 activates pro-MMP-3 but not pro-MMP-1. ( a ) We evaluated the cysteine protease activity of WT-r-CP-A5 and C119S-r-CP-A5 using a specific fluorescence substrate (ZRR-AMC). No cysteine protease activity was observed with immature proteases (pro-WT-r-CP-A5 and pro-C119S-r-CP-A5). The WT-r-CP-A5 possesses proteolytic activity but this was very low in the C119S mutant. ( b , c ) We measured MMP activities using the MMP-specific substrate FS-6 specific. ( b ) Pro-MMP-1 and [MMP-1:TIMP-1] complex was incubated with either WT-r-CP-A5 or C119S-r-CP-A5 but was never activated. ( c ) Pro-MMP-3 was specifically activated by the mature WT-CP-A5. This activation required the enzymatic activity of CP-A5. Interestingly, MMP-3 activated by WT-r-CP-A5 can in turn convert pro-MMP-1 (arrow heads) into its mature form. Results are shown as mean and the s.d. Data are shown as mean and the s.d. The data are from six independent experiments, n =6. Nonparametric Mann–Whitney test was performed, * P <0.05. A.U. : arbitrary units. Full size image We also measured the in vitro activity of both pro-MMPs-1 and -3 using peptide FS-6, a highly specific fluorescent substrate for MMPs [18] . In the presence of the chemical activator 4-aminophenylmercuric acetate (APMA), we measured a strong increase in the fluorescence, thereby confirming that MMPs-1 and -3 were enzymatically active after APMA treatment ( Supplementary Fig. 1B,C ). We also demonstrated that pro-MMP-1, pro-MMP-3, the [MMP-1:TIMP-1] and [MMP-3:TIMP-1] complexes, and WT-r-CP-A5 were not able to cleave the FS-6 substrate; any increase in fluorescence was thus specific for activated MMPs. We then incubated activated WT-r-CP-A5 or activated C119S-r-CP-A5 with pro-MMP-1, pro-MMP-3 and the [MMP-1:TIMP-1] or [MMP-3:TIMP-1] complex ( Fig. 7b,c ). Neither WT-r-CP-A5 nor C119S-r-CP-A5 activated pro-MMP-1 or the [MMP-1:TIMP-1] complex ( Fig. 7b ). We never observed MMP-3 activation when it was complexed with TIMP-1. In contrast, the increase in fluorescence when WT-r-CP-A5 was incubated with pro-MMP-3 indicated that WT-r-CP-A5 activates pro-MMP-3 into its mature form. This activation of pro-MMP-3 was not observed in the presence of C119S-r-CP-A5 ( Fig. 7c ). Taken as a whole, these results demonstrate that the cleavage of pro-MMP-3 relies on the enzymatic capabilities of CP-A5. Interestingly, the addition of pro-MMP-1 to the enzymatic reaction containing WT-r-CP-A5 and pro-MMP-3 was associated with an increase in fluorescence (reflecting an increase in MMP activity). These results indicate that in vitro , WT-r-CP-A5 activates pro-MMP-3 into its mature form, which in turn activates pro-MMP-1. WT-CP-A5 restores invasion of CP-A5-silenced strain To confirm the key role of CP-A5 proteolytic activity during intestinal invasion, we added either WT-r-CP-A5 or C119S-r-CP-A5 to CP-A5-silenced trophozoites. As a control, we compared the invasive ability of CP-A5-deficient trophozoites with the invasive ability of Amoebapore-A-silenced trophozoites (G3 strain). After 7 h of contact with trophozoites, colon fragments were prepared for histological analysis and longitudinal sections of the tissue were analysed ( Fig. 8a ). CP-A5-silenced trophozoites complemented with WT-r-CP-A5 were rescued for their invasive phenotype; they invaded the colonic mucosa to the same extent as the WT and G3 strain. In contrast, CP-A5-silenced trophozoites incubated with C119S-r-CP-A5 were not rescued and did not invade the mucosa; hence, CP-A5 proteolytic activity in situ is essential for intestinal invasion. Taken as a whole, these data indicate that upon intestinal invasion, CP-A5 induces a cascade of MMPs-3 and -1 activation, fibrillar collagen remodelling and subsequent mucosa invasion. Quantification of tissue invasion for each condition is shown in Fig. 8b . 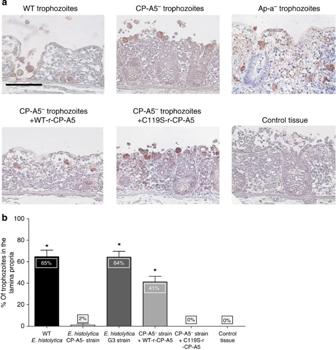Figure 8: Purified WT-r-CP-A5 restores the defective phenotype of CP-A5-silenced strain. Human colon explants were incubated for 7 h with WT, Amoebapore-A-silenced trophozoites and CP-A5-silenced trophozoites, and WT-r-CP-A5 or C119S-r-CP-A5 were added to the incubation medium. (a) After tissue treatment for histology, trophozoites were immunohistochemically stained for Gal/GalNAc lectin and counterstained with haematoxylin–eosin. Addition of C119S-r-CP-A5 to CP-A5-silenced trophozoites did not restore an invasive phenotype. Trophozoites were not able to invade the lamina propria and were observed at the surface of the explant (as were CP-A5-silenced trophozoites alone). However, incubation of CP-A5-silenced trophozoites with WT-r-CP-A5 restore the invasive phenotype. Trophozoites were present in the lamina propria (as seen with the WT strain and Amoebapore-A-silenced trophozoites). One representative image of the three experiments performed is shown. Scale bar, 50 μm.n=3. (b) For each condition, trophozoites present in the lamina propria were quantified. Data are shown as mean and the s.d. of the mean. The data are from three independent experiments (n=3). Nonparametric Mann–Whitney test was performed. *P<0.05. Figure 8: Purified WT-r-CP-A5 restores the defective phenotype of CP-A5-silenced strain. Human colon explants were incubated for 7 h with WT, Amoebapore-A-silenced trophozoites and CP-A5-silenced trophozoites, and WT-r-CP-A5 or C119S-r-CP-A5 were added to the incubation medium. ( a ) After tissue treatment for histology, trophozoites were immunohistochemically stained for Gal/GalNAc lectin and counterstained with haematoxylin–eosin. Addition of C119S-r-CP-A5 to CP-A5-silenced trophozoites did not restore an invasive phenotype. Trophozoites were not able to invade the lamina propria and were observed at the surface of the explant (as were CP-A5-silenced trophozoites alone). However, incubation of CP-A5-silenced trophozoites with WT-r-CP-A5 restore the invasive phenotype. Trophozoites were present in the lamina propria (as seen with the WT strain and Amoebapore-A-silenced trophozoites). One representative image of the three experiments performed is shown. Scale bar, 50 μm. n =3. ( b ) For each condition, trophozoites present in the lamina propria were quantified. Data are shown as mean and the s.d. of the mean. The data are from three independent experiments ( n =3). Nonparametric Mann–Whitney test was performed. * P <0.05. Full size image In the present study, we investigated the relationship between CP-A5 and human MMPs during intestinal amoebiasis. Given that human MMPs are known to be responsible for degrading ECM in connective tissue [11] and are tightly controlled by inflammatory cytokines, we hypothesized that human MMPs are involved in the destruction of the ECM of the lamina propria during intestinal invasion by E. histolytica . This hypothesis was supported by the fact that CP-A5 induces secretion of TNF-α and IL-1β (ref. 8 ), which in turn can induce MMP expression. Using human colon explants, we determined that MMP enzymatic activity is responsible for the alteration of fibrillar collagen structures present in the lamina propria during intestinal invasion by E. histolytica . We observed the specific overexpression of MMPs-1 and -3 genes during intestinal invasion in agreement with clinical data obtained from patient biopsies [10] . We demonstrated that this phenomenon was dependent on the presence of CP-A5. In the presence of marimastat, ECM degradation is abolished preventing the formation of ECM-derived bioactive molecule [19] , [20] and consequently reducing activation of resident immunes cells. In situ immunofluorescence and western blot analysis confirmed that the expression and activation of MMPs-1 and -3 was dependent on the presence of CP-A5. Interestingly, it has been shown that pro-CP-A5 contains a Arg-Gly-Asp ( RGD ) motif that can bind directly to α ν β 3 integrin on colon epithelial cells and triggers integrin/NFκB (nuclear factor κB) signalling, which in turn elicits pro-inflammatory cytokine production (TNF-α and IL-1β; ref. 8 ). This intriguing mechanism does not require CP-A5 enzymatic activity [8] . The MMP genes are transcriptionally responsive to TNF-α (refs 21 , 22 ) and IL-1β (refs 9 , 23 , 24 , 25 ). Functional experiments in an ex vivo human fetal small intestine explant model have clearly shown that MMP-3 acts as a key molecule of TNF-α-mediated tissue injury in the gut [26] , [27] . In our model, we saw that by inducing TNF-α and IL-1β (ref. 8 ) secretion, pro-CP-A5 stimulated MMPs-1 and -3 expression and mediated collagen remodelling during the invasion of the lamina propria. As MMPs can be released as inactive forms (either as the immature pro-form or complexed with TIMPs), we looked at whether CP-A5’s proteolytic activity could activate human MMPs. After the co-incubation of MMPs-1 and -3 with recombinant CP-A5, we observed that mature CP-A5 was able to convert pro-MMP-3 into the active catalytic enzyme. Furthermore, we demonstrated that pro-MMP-1 is not directly activated by mature CP-A5; in fact, CP-A5 activates pro-MMP-3, which in turn activates pro-MMP-1. Stromelysin-1 (MMP-3) cleaves proteoglycans, collagen (types II, IX and XI), gelatin, laminin and fibronectin, and has been linked to tissue degradation in pathological situations (such as inflammatory bowel disease and Crohn’s disease) in which MMP-3 contributes to ECM degradation [28] , [29] . In our disease model, MMP-3 was expressed by epithelial cells, suggesting that this enzyme could contribute to extensive desquamation through degradation of the basal membrane, which supports the epithelial cells lining in the colon. Another interesting role of MMP-3 relates to its ability to activate pro-MMP-1 (ref. 12 ). In turn, activated MMP-1 is then able to directly perform the intrahelix cleavage of native fibrillar collagen within the ECM [13] , [14] . Given that (i) fibrillar collagen fibres cleaved by collagenase were observed during invasion of the mucosa and (ii) active MMP-3 was also present, we hypothesize that MMP-1 is active and involved in ECM remodelling. Moreover, since CP-A5-silenced trophozoites were able to regain their invasive phenotype when complemented by the recombinant WT-CP-A5, we speculate that the MMP-3/MMP-1 activation cascade occurs in situ and is triggered by CP-A5 proteinase activity. In conclusion, we propose a two-step mechanism in which CP-A5 collaborates with MMPs to induce ECM remodelling during intestinal invasion ( Fig. 9 ). First, upon contact with epithelial cells, pro-CP-A5 elicits the secretion of pro-inflammatory cytokines (TNF-α and IL-1β), which in turn trigger the synthesis and expression of MMPs-1 and -3. This initiation of the host pro-inflammatory response constitutes CP-A5’s signalling role at early stages of the invasive process. Second, CP-A5 catalytically cleaves pro-MMP-3 into the active enzyme, which in turn activates other MMPs (including MMP-1) and then degrades ECM. It is noteworthy that trophozoites secrete both pro-CP-A5 and mature form [30] , which thus potentially induces and activates human MMPs at the same time. Together, the combined actions of CP-A5 contribute to the ECM destruction by human MMPs and to the acute inflammation observed during intestinal amoebiasis. 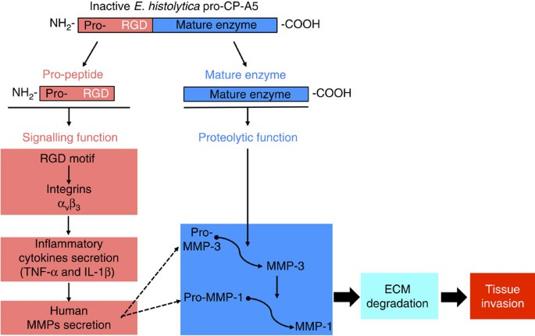Figure 9: The dual role of CP-A5 during intestinal invasion. Our working model considers two step to explain how CP-A5 collaborates with MMPs to induce ECM remodelling during intestinal invasion. First, pro-CP-A5 (containing the RGD motif) triggers at early stages of invasion the secretion of pro-inflammatory cytokines through integrin signalling (and thus inducing human MMP synthesis and release). Second, mature CP-A5 cleaves pro-MMP-3 into active MMP-3, which is then able to activate pro-MMP-1. Finally, the active MMPs degrade ECM components and allow mucosa invasion byE. histolyticatrophozoites. Figure 9: The dual role of CP-A5 during intestinal invasion. Our working model considers two step to explain how CP-A5 collaborates with MMPs to induce ECM remodelling during intestinal invasion. First, pro-CP-A5 (containing the RGD motif) triggers at early stages of invasion the secretion of pro-inflammatory cytokines through integrin signalling (and thus inducing human MMP synthesis and release). Second, mature CP-A5 cleaves pro-MMP-3 into active MMP-3, which is then able to activate pro-MMP-1. Finally, the active MMPs degrade ECM components and allow mucosa invasion by E. histolytica trophozoites. Full size image Patient samples Healthy segments of human colon were obtained from patients undergoing colon surgery at Foch Hospital (Suresnes, France). The patients provided their written informed consent for use of the samples in the present study. The data were analysed anonymously at the Pasteur Institute. Tissues were processed in accordance with the French government’s guidelines for research on human tissues and the French Bioethics Act. The study protocol was approved by a regional investigational review board (Comité de Protection des Personnes, Ile de France VII, Paris, France) and an institutional review board (Institut Pasteur Recherche Biomedicale, Paris, France; reference RBM/2009.50). Parasite cultures The pathogenic E. histolytica strain used in this study was HM1:IMSS. This virulent strain was also used to produce trophozoites epigenetically silenced for Amoebapore A (strain G3) or CP-A5 (strain RB8; refs 31 , 32 ). Trophozoites were grown axenically in TYI-S-33 medium at 37 °C. All trophozoites were harvested during the exponential growth phase and collected by centrifugation at 300 g for 5 min. Human colon explant preparation and histological analysis The resected tissues were dissected under a stereomicroscope in order to remove fat and muscle and to retain the mucus, the mucosa and the submucosa. The explant were cut into segments measuring 3 cm by 1.5–2 cm (that is, 5.5–6 cm 2 ) and pinned (with the submucosa facing down) onto 4% agarose layer in tissue culture dishes (60 × 20 mm; Schott Duran, Germany). Trophozoites (8 × 10 5 in 1 ml of Krebs medium) were added to the luminal face of the colon and incubated in Krebs buffer at 37 °C in the presence or absence of marimastat (200 nM; Sigma-Aldrich). After 7 h of incubation, tissue fragments were fixed in paraformaldehyde (4%) and included in paraffin. Paraformaldehyde-fixed tissue sections were then processed for immunohistochemistry. The trophozoites were immunostained with a 1/200 diluted rabbit serum raised against the Gal/GalNAc lectin [3] . For each experiment, a representative histology image was shown. Quantification of human colon invasion Human colon invasion by E. histolytica was quantified by counting on transverse histological slice 100 trophozoites immunostained against the Gal/GalNAc lectin (brown). Images were obtained using a light microscope (Nikon, Eclipse E800). Then the percentage of trophozoites inside the lamina propria (for example, below the epithelial monolayer) was determined. Values correspond to the mean (±s.d.) of four experiments performed. Collagen degradation assays E. histolytica WT, trophozoites were resuspended in TYI media (3 × 10 5 trophozoites per millilitres) and then incorporated into a bovine collagen I solution (1.7 mg ml −1 ) containing 2% DQ FITC (fluorescein isothiocyanate)-labelled type I collagen monomers (Invitrogen, Molecular Probes). Marimastat (200 nM) was added to the collagen lattice before polymerization and trophozoites were pretreated for 30 min before incorporation. After 0, 6 and 24 h of culture at 37 °C, solid-phase collagen was pelleted (5 min, 16,000 g ) and the supernatant containing released fluorescein isothiocyanate–collagen fragments was measured spectrofluorimetrically (Fluoroskan Ascent, ThermoLabsystems, 480 nm excitation and 520 nm detection). The background signal and total degradation were obtained from a cell-free lattice (basal level) and in the presence of type VII collagenase from Clostridium histolitycum (7 U ml −1 , 6 h, 37 °C; positive control), respectively. Four experiments were performed and data are shown as mean of fluorescence values (±s.d.). Multiphoton (MPM) and second-harmonic generation imaging microscopy (SHIM) Trophozoites were labelled using a CellTracker Green CMFDA or CellTracker Red CMTPX (Molecular Probes, Invitrogen). For multiphoton (MPM) and SHIM, we used a laser-scanning microscope (LSM710 Meta, Zeiss, Germany) with a TI: sapphire femtosecond laser (140 fs, 90 MHz) that was tunable from 690 to 1,040 nm (Cameleon ultra I, Coherent), together with a Zeiss Plan-APOCHROMAT × 20 objective (1 numerical aperture water immersion). The excitation wavelength was 820 nm. The detection bandwidths were 500–550 nm (pseudocoloured purple) and 570–610 nm (pseudocoloured red) for MPM, and 400–420 nm (pseudocoloured green) for SHIM. Signals were collected with a backscattering geometry and were not descanned. The Zen 2008 SP 1.1 software package (Zeiss) and LSM Image Browser (Zeiss) were used to acquire and prepare images, respectively. RNA isolation, cDNA synthesis and qRT–PCR analysis RNA was directly isolated from FFPE tissue using the RNEasy FFPE kit (Qiagen). Total RNA quantity and purity were determined by optical density at 260 and 280 nm by using a spectrophotometer. The RNA samples were treated with DNAse I Amp Grade (Invitrogen). The absence of genomic DNA contamination was confirmed by using the treated RNA as a template in PCRs. One microgram of total RNA was used for a reverse transcription reaction with Oligo(dt) 12–18 primers and SuperScript II reverse transcriptase (SuperScript first-strand synthesis system for RT–PCR, Invitrogen) for the evaluation of relative expression. Negative controls were set up by replacing the reverse transcriptase with RNAase-free water. The resulting single-stranded cDNA was then used for qRT–PCR analysis (ABI PRISM 7900HT) to evaluate relative expression. cDNA was combined with primer/probe sets and IQ SYBR Green Supermix (Bio-Rad), according to the manufacturer’s recommendations. All primers were validated at http://pga.mgh.harvard.edu/primerbank/ ( Table 1 ) and purchased from Invitrogen. The PCR conditions were 95 °C for 3 min, followed by 45 cycles with denaturation at 95 °C for 15 s, annealing temperature for 30 s and elongation at 72 °C for 30 s. The PCRs’ specificity was assessed by analysing the melting curves. To normalize the amount of cDNA, we sampled equal amounts of quantified RNA, assessed its quality before reverse transcription and used reference genes for comparison. Fold change were calculated using the average cycle threshold for the glyceraldehyde-3-phosphate dehydrogenase and ribosomal protein L13 genes in each tissue. Table 1 Primer used in quantitative PCR experiments. Full size table Immunofluorescence and confocal microscopy analysis Five-micron FFPE tissue sections were dewaxed and rehydrated with serial alcohol solutions. To retrieve antigens, sections were heated at 95 °C for 1 h in a 10-mM sodium citrate solution and allowed to cool to room temperature. Sections were incubated in 1% PBS/bovine serum albumin (Sigma-Aldrich) for 1 h at room temperature (to avoid nonspecific labelling) and were incubated overnight with the corresponding primary antibody: MMP-1 (1:100 dilution; sc-21731; Santa Cruz Biotechnology), MMP-3 (1:200; ab53015; Abcam, Cambridge, UK), MMP-9 (1:200, sc-6840; Santa Cruz Biotechnology). The COL 2 3/4C (1:100; 50-1035; IBEX Pharmaceuticals Inc., Canada) short antibody detects collagenase-cleaved type I and II collagen. More specifically, it recognizes the α-chain fragments containing an ~8 amino-acid sequence at the carboxy terminus of the three-quarter piece produced by collagenase (MMPs-1, -8 and -13) cleavage of type I and II collagen. Sections were washed in PBS and incubated with fluorescently labelled Alexa Fluor 594 goat anti-rat (1:400; A-11007) or Alexa Fluor 488 goat anti-rabbit (1:400; A-11008) secondary antibodies (Molecular Probes, USA) and 4',6-diamidino-2-phenylindole to visualize nuclei. The sections were washed and the slides were then mounted using VectaShield mounting medium and sealed with nail polish. The slides were analysed using a Zeiss LSM710 scanning-laser confocal microscope and LSM ZEN software. A three-laser beam (350, 488 and 568 nm) was used for excitation of the fluorophores, using a × 25 Plan-NEOFLUAR oil immersion lens (0.8 numerical aperture). Immunofluorescence staining experiments were repeated in triplicate with multiple serial sections (including a negative control for determining background staining). Recombinant expression, refolding and processing of CP-A5 Recombinant expression of Wt-r-CP-A5 or the C119S-r-CP-A5 was performed as previously described [33] and was carried out by GenScript USA Inc. (Piscataway Township, NJ, USA). In brief, the gene encoding the pro-form of EhCP5 (accession number: EHI_168240; amino-acid residues 14–317) was synthetized and cloned into pUC57 (encoding a 10-residue histidine tail that is added to the gene product at the N terminus). Escherichia coli (BL-21 strain) were transformed with recombinant plasmids. The bacteria were induced and proteins were obtained from inclusion bodies after purification on a nickel column. Proteins were eluted and the concentration was determined in a Bradford protein assay with bovine serum albumin as a standard. Aliquot fractions were analysed on an SDS–polyacrylamide gel electrophoresis gel. Densitometry analysis suggested a purity of ~85%. Recombinant CP-A5 was refolded as described [33] , and CP-A5 was processed into enzymatically active protein by incubation in a buffer containing 0.08% SDS, 10 mM DTT, 100 mM Tris-HCl, pH 8.8, at 37 °C for 60 min. Protease activation and transactivation experiments CP-A5 proteolytic activity with the synthetic peptides ZRR-AMC (Bachem) was determined as described [34] . Specific enzymatic activity was expressed in micromoles of released fluorescent substrate per minute per milligrams of recombinant protein. MMPs-1 and -3 (R & D SYSTEMS EUROPE) proteolytic activity was determined using the substrate FS-6 (Sigma-Aldrich; excitation: 325 nm and emission: 400 nm; ref. 18 ). For MMP activation, purified pro-MMPs-1 and -3 were diluted to 50 μg ml −1 in assay buffer (50 mM Tris, 10 mM CaCl 2 , 150 mM NaCl and 0.05% Brij-35, pH 7.5). APMA (1 mM) was used as a chemical activator and TIMP-1 (1:1 ratio) (R & D SYSTEMS EUROPE) was used to inhibit the mature form after 2 h of incubation. Activated recombinant WT-r-CP-A5 and C119-r-CP-A5 enzymes were incubated with pro-MMP-1, pro-MMP-3, the [MMP-1:TIMP-1] or [MMP-3:TIMP-1] complexes for 2 h in assay buffer. Finally, the MMPs were diluted to 1 ng μl −1 and 50 μl were mixed with 50 μl of FS-6 (20 μM). MMP activation was recorded by monitoring emission at 400 nm (Infinite 200 PRO ). Statistical analysis Data (from protease activity or qPCR experiments) were independent and non-normally distributed, the Mann–Whitney test was selected for the statistical analysis using GraphPad Prism software (version 3.00, GraphPad Software Inc., San Diego, CA, USA). The threshold for statistical significance was set to P <0.05. (* P <0.05; NS, not significant P ≧ 0.05). How to cite this article: Thibeaux, R. et al. The parasite Entamoeba histolytica exploits the activities of human matrix metalloproteinases to invade colonic tissue. Nat. Commun. 5:5142 doi: 10.1038/ncomms6142 (2014).